Discovery of lost diversity of paternal horse lineages using ancient DNA Modern domestic horses display abundant genetic diversity within female-inherited mitochondrial DNA, but practically no sequence diversity on the male-inherited Y chromosome. Several hypotheses have been proposed to explain this discrepancy, but can only be tested through knowledge of the diversity in both the ancestral (pre-domestication) maternal and paternal lineages. As wild horses are practically extinct, ancient DNA studies offer the only means to assess this ancestral diversity. Here we show considerable ancestral diversity in ancient male horses by sequencing 4 kb of Y chromosomal DNA from eight ancient wild horses and one 2,800-year-old domesticated horse. Both ancient and modern domestic horses form a separate branch from the ancient wild horses, with the Przewalski horse at its base. Our methodology establishes the feasibility of re-sequencing long ancient nuclear DNA fragments and demonstrates the power of ancient Y chromosome DNA sequence data to provide insights into the evolutionary history of populations. The Y chromosome is a valuable tool in population genetics, as it provides a means to directly assess evolutionary processes that only affect the paternal lineage. The use of Y chromosome data in population genetic analyses became widely established in reconstructions of human evolutionary relationships and demographic processes (for a review see ref. 1 ). However, very few Y chromosome studies have focused on non-model taxa. This may in part be due to challenges associated with developing Y chromosomal markers which include a proliferation of repeat elements and the low genetic diversity characteristic of the Y chromosome [2] . In a recent comparative analysis of five mammalian species, two (wolf and field vole) show low levels of nucleotide diversity on the Y chromosome (π Y 0.4×10 −4 and 1.7×10 −4 , respectively), while the other three (lynx, reindeer and cattle) had no diversity at all [3] . Low Y chromosomal genetic diversity was also observed in sheep [4] , cattle [3] , [5] and dogs [6] , [7] . These results suggest a general pattern of low male effective population size in domestic mammals, which may be attributable to breeding practices associated with domestication, where few males are selected to mate with a wider variety of females. One of the most extreme examples of contrasting levels of genetic diversity between maternal and paternal markers is the domestic horse. Using microsatellite data [8] and up to 14.3 kb of sequence data from 52 individuals representing 15 breeds, all but one investigation has failed to detect any diversity on the Y chromosome of modern horses [8] , [9] , [10] , [11] . In the study that did detect diversity, a single polymorphic microsatellite was reported from a sample of domestic Chinese horses [12] . In contrast, the maternally inherited mitochondrial genome shows abundant diversity both among and within horse breeds with limited, to no, correlation between breeds and mitochondrial DNA haplotypes [13] , [14] , [15] , [16] , [17] . Several hypotheses have been proposed to explain the contrasting mitochondrial and Y chromosome diversity in domestic horses. First, the number of domestic founders may have differed between the sexes, with a small number of males (low male effective population size) [8] , [9] , [10] , [11] and a larger number of females, the latter possibly originating from multiple geographical regions [14] , [15] . Second, reproductive success among males may be strongly skewed because of the naturally polygamous mating system of horses [18] , [19] or resulting from a breeding scheme imposed by humans during or after domestication, where a few select studs were preferentially mated with many mares [20] , [21] . Third, as generally suggested for uniparentally inherited sex chromosomes [3] , selection may have eliminated genetic diversity on horse Y chromosomes due to either purifying background selection or selective sweeps caused by positive selection. These hypotheses are not mutually exclusive, and multiple forces may have operated together to eliminate variability on the domestic horse Y chromosome. Unfortunately, almost no wild horses remain; the only surviving wild horse population is a small captive stock of Przewalski horses, which represent the closest living relatives of domesticated horses. Notably, Przewalski horses experienced an extreme population bottleneck during the last century; the captive stock was founded by only eight females and five males, and hybridization with domesticated horses cannot be excluded [22] . Therefore, DNA amplified from ancient remains provides the only means to investigate the extent and nature of the genetic diversity of wild horses. Thus far, this approach has been used only for mtDNA [13] , [14] , [16] , [23] , [24] , [25] the results of which suggest that domestication was not a significant bottleneck for horse mtDNA diversity [26] . Consequently, high mtDNA diversity in domestic horses has been explained by high diversity of the founding population, multiple origins of domestication, further domestication events during the Iron Age, and backcrossing with wild mares from different populations. In contrast to mtDNA, the technical challenges associated with large-scale targeted re-sequencing of ancient nuclear DNA have so far prevented studies of the Y chromosomal diversity of past horse populations. For example, the high copy-number of mtDNA per cell has facilitated its use in ancient DNA analyses, as the probability that fragments survive over time is greater simply because of the larger number of starting molecules. It has recently been shown that the ratio of autosomal DNA to mtDNA increases from ∼ 1:152 in modern tissues to 1:245–17,480 in ancient tissues, most likely owing to differential preservation [27] . For the Y chromosome, this ratio decreases by another factor of two. In addition to fewer starting molecules, the expected low diversity in the Y chromosome means that longer regions of the Y chromosome need to be sequenced to observe sufficient polymorphisms for analysis. Further, Y chromosomes can only be found in the remains of male individuals, and the sex of the remains is generally unknown. In this study, we successfully amplified 4 kb of Y chromosome DNA from nine ancient horse specimens, including one 2,800-year-old domesticated horse. This represents the first ancient Y chromosome re-sequencing dataset to date. Using these data, we investigated Y chromosome diversity in pre-domestication ancient wild-horse populations, and compared the results with what is known about Y-chromosome diversity in modern domestic and Przewalski's horses. We found that the ancient horses harboured considerable Y-chromosome diversity. 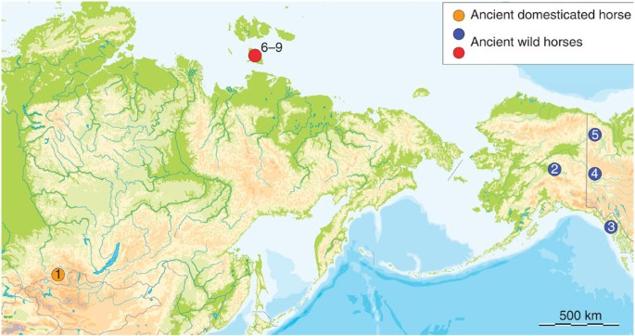Figure 1: Geographic origin of the ancient horse samples. The continental-scale origin of the ancient wild horses is further emphasized in red (Eurasia) and blue (North America). Sample Abbreviations: 1=ARZ-1-3, 2=JAL-292, 3=JAL-310, 4=YG 109.6, 5=MGVo1_niche3.3, 6=BL-O485,7=BL-O250, 8=BL-O728, 9=ML-O112. Sequencing of ancient DNA We sequenced a total of 4,062 bp of Y-chromosomal DNA from each of eight wild horses from permafrost sites in Siberia and North America, and one 2,800-year-old domestic stallion (see Table 1 and Fig. 1 ). Including the six sites that differ between modern Przewalski's horse and modern domestic horses, we identified 28 segregating sites among all sequenced horses ( Supplementary Table S1 ). 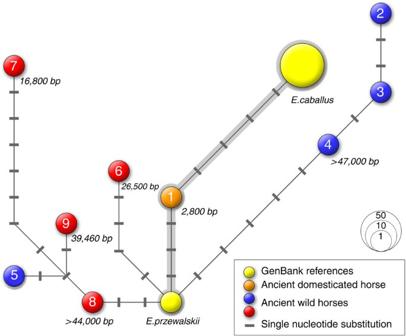Figure 2: Median-Joining network based on 4,062 bp Y chromosomal sequence. The continental-scale origin of the ancient wild horses is shown by different colours (red: Eurasia; blue: North America). The 2,800-year-old domestic horse haplotype is shown in orange and sequences retrieved from NCBI GenBank in yellow. Haplotypes sharing the 4bp deletion are shaded in grey. Sample Abbreviations:1=ARZ-1-3, 2=JAL-292, 3=JAL-310, 4=YG 109.6, 5=MGVo1_niche3.3, 6=BL-O485,7=BL-O250, 8=BL-O728, 9=ML-O112. Each of our ancient horses carried a unique haplotype with pairwise sequence differences among individuals ranging from 1 to 16 substitutions ( Table 2 ). All sequence positions were replicated at least twice, excluding ancient DNA damage as a possible cause for the polymorphic positions observed. Nucleotide diversity (π Y ) was estimated to be 1.89×10 −3 (standard deviation (s.d.) 3.00×10 −4 ) in the wild horses including the Przewalski horse. Since nucleotide diversity was found to be zero in modern domestic horse Y chromosome sequences [10] , and because demographic processes between the timing of domestication and today remain unknown, it is not possible to accurately estimate π Y for domestic horses. As an approximation, we calculated π Y for modern domestic horses plus the single ancient domestic haplotype sequenced as part of this study to be 4.00×10 −5 (s.d. 4.00×10 −5 ). Table 1 Information about the ancient samples amplified for the full 4 kb Y chromosomal DNA sequence. Full size table Figure 1: Geographic origin of the ancient horse samples. The continental-scale origin of the ancient wild horses is further emphasized in red (Eurasia) and blue (North America). Sample Abbreviations: 1=ARZ-1-3, 2=JAL-292, 3=JAL-310, 4=YG 109.6, 5=MGVo1_niche3.3, 6=BL-O 485 ,7=BL-O 250 , 8=BL-O 728 , 9=ML-O 112 . Full size image Table 2 Number of pairwise nucleotide differences among all horse sequences. Full size table Phylogenetic relationship of Y chromosome haplotypes The phylogenetic relationship among all 62 available horse Y chromosome haplotypes (nine from our study plus 52 modern horses and the Przewalski horse haplotype from ref. 10 ) is depicted in a median joining network ( Fig. 2 ). The haplotype of the 2,800-year-old domestic horse is most similar to that of modern horses, differing by four substitutions. The ancient horses cluster into three branches in the network: one consists exclusively of North American samples, one consists of a single Siberian sample, and the third one shares haplotypes from both North America and Siberia but is dominated by Siberian haplotypes. The Przewalski horse is basal to the domestic lineage, and shares a 4-bp deletion with domesticated horses that is not found in any ancient wild horse. Figure 2: Median-Joining network based on 4,062 bp Y chromosomal sequence. The continental-scale origin of the ancient wild horses is shown by different colours (red: Eurasia; blue: North America). The 2,800-year-old domestic horse haplotype is shown in orange and sequences retrieved from NCBI GenBank in yellow. Haplotypes sharing the 4bp deletion are shaded in grey. Sample Abbreviations:1=ARZ-1-3, 2=JAL-292, 3=JAL-310, 4=YG 109.6, 5=MGVo1_niche3.3, 6=BL-O 485 ,7=BL-O 250 , 8=BL-O 728 , 9=ML-O 112 . Full size image Incorporating temporally sampled data may artificially increase observed diversity, if the mutation rate is fast relative to the temporal span of the sequences. Although the ancient horses investigated lived during different time periods (ranging from >47 ky–2.8 ky years, Table 1 ), the temporal distribution of our samples does not seem to inflate our diversity estimates, as no correlation appears between the number of pairwise substitutions and the age of the samples (Spearman correlation coefficient, P -values based on exact matrix permutation: r =−0.033, P =0.942). This pattern is maintained after swapping the dates of the two infinitely dated samples ( r =−0.152, P =0.658). Further, we performed a molecular-clock based phylogenetic analysis both to estimate the age of the most recent common ancestor of all of the Y chromosome haplotypes and to determine when the various lineages diverged ( Fig. 3 ). The time to the most recent common ancestor of all Y chromosomal horse haplotypes is 92–380 ka bp, with a mean of 208 ka bp. The shape of the MCMC genealogy indicates that most of the Y chromosome lineages emerged before the age of the oldest sample (53,800 years BP ). As only two Y chromosome lineages persist today (the modern domestic lineage and the Przewalski lineage) this suggests a significantly higher diversity in the past. 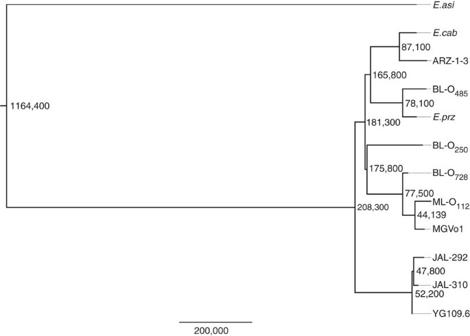Figure 3: Chronogram of horse Y chromosome evolution. Topologies and divergence time estimates (node labels) for the respective branches were inferred using BEAST v1.6.0 (refs51,52) under the settings described in the main text. One donkey (E.asinus) sequence was used as an outgroup. Figure 3: Chronogram of horse Y chromosome evolution. Topologies and divergence time estimates (node labels) for the respective branches were inferred using BEAST v1.6.0 (refs 51 , 52 ) under the settings described in the main text. One donkey ( E.asinus ) sequence was used as an outgroup. Full size image The relationship of Przewalski's horse to modern domestic horses remains controversial [9] , [11] , [17] , [28] , [29] , [30] . Przewalski horses are generally viewed as either the last surviving wild-horse population, or a feral-horse population derived from a primitive domestic lineage. The issue is confounded by a recent population bottleneck [22] that is likely to have reduced the genetic diversity within Przewalski horses significantly. Today, two mtDNA haplotypes are found in Przewalski horses, and neither of these is present in modern horses. It has been proposed therefore that Przewalski horses are not ancestral to modern domestic horses [23] , [30] . However, the Przewalski haplotypes do fall within the large diversity of modern horse mtDNA [14] , [15] , [17] , [25] . A similar pattern was shown for autosomal DNA [11] , [31] and X chromosomal sequences [11] , where it was not possible to separate the Przewalski horses phylogenetically from domestic horses, although differences in the autosomal and X chromosomal nucleotide diversity in both taxa indicate a different evolutionary history [11] . Our results indicate that the single Przewalski's horse Y chromosome haplotype [9] , [10] falls within the greater Y chromosomal diversity of domestic and ancient wild horses. Interestingly, the Przewalski Y chromosome haplotype is more closely related to the two domestic horse haplotypes in our data set than any of the ancient wild horses. Thus, in agreement with the other genetic markers, the Y chromosome data presented here supports historic isolation, but, at the same time, a close evolutionary relationship between domestic horse and Przewalski's horse. All 52 domestic horses that have been sequenced to date, representing 15 modern horse breeds, have identical Y chromosome haplotypes [10] . One hypothesis to explain this suggests that modern horses have little Y chromosome diversity because the wild horses from which they were domesticated were also not diverse, due in part to the harem mating system in horses, implying skewed reproductive success of males [19] . Our results reject this hypothesis, suggesting instead that the Y chromosome diversity estimated from ancient wild horses (π Y 1.89×10 −3 ) is high, and particularly high in comparison to that estimated previously for other wild mammals (for example, European rabbit π Y 1.34×10 −3 (ref. 32 ), wild boar π Y 0.98×10 −3 (ref. 33 ), felidae π Y 0–0.995×10 −3 (ref. 34 ) and wolf π Y 0.04×10 −3 (ref. 3 ). Although it is difficult to directly compare absolute values of diversity among different species, these numbers show that ancient wild horses harboured substantial genetic diversity on the Y chromosome. Because we sample over a window of time rather than within a single time-frame, the diversity measurements may be artificially inflated if new mutations arise during the sampling period. However, the age range of the samples from which our data are derived is small relative to the mutation rate of the Y chromosome. We therefore expect few if any novel mutations to arise during this period, and little influence on the diversity estimate. The abundant Y chromosomal diversity found in wild horses is in stark contrast to the complete lack of variability in modern horses. This result argues against the absence of Y chromosomal diversity in modern horses being based on properties intrinsic to wild horses, such as continuous strong selection on the Y chromosome or a strong reproductive skew among males. Our results therefore support the hypothesis that the lack of genetic diversity in extant horses may be a consequence of the domestication process. This loss of diversity at domestication may have been achieved either through the incorporation of very few wild male horses in the domestic stocks [8] , [9] , [10] , [11] , a global selective sweep of the Y chromosome [8] , or breeding practices developed after domestication that reduced the effective number of males in the domestic species [20] , [21] . The first hypothesis predicts that low levels of Y chromosome diversity will be found in all historic and prehistoric domestic horses. The second and third hypotheses both predict high Y chromosome genetic diversity in early domestic horses followed by a decrease to modern/near the modern very low level of diversity. The single, domesticated horse sequence in our data set originates from a Scythian tomb and dates to 2,800 years BP . Artefacts recovered from the same site from which the specimen originates have been associated with riding, and show direct evidence of domestication [35] . This sample shows a haplotype that is closely related to, but distinct from the modern haplotype, from which it differs by four substitutions. Given the relatively young age of the sample and the estimated substitution rate of 0.85% per million years, it is unlikely that the haplotype found in the Scythian horse is a direct ancestor of the haplotype that characterizes all sequenced modern horses. Although data from a single ancient domesticated horse is not conclusive, it does show that more genetic variation existed within domestic horses 2,800 years ago than which exists today. However, the single sample cannot distinguish between breeding practices or a global selective sweep as the cause of the eventual complete loss of genetic diversity in domestic horses. To characterize both the initial level of Y chromosomal diversity in domestic horses and the processes by which this was lost, it will be necessary to obtain data from both early domestic horses, such as those from Botai [36] , [37] , as well as from later periods such as the Iron age or Medieval times, ideally in combination with mitochondrial and autosomal sequence data. So far, ancient DNA studies comparing homologous, replicated sections of DNA from multiple individuals have been mostly limited to mitochondrial DNA. Although nuclear DNA sequences from three Neanderthal specimens have been published recently [38] , these were obtained by low coverage shotgun sequencing, an approach that is not generally scalable to address population genetic questions. However, our results show that by using a regular two-step multiplex PCR, it is possible to obtain nuclear and even Y chromosomal DNA data sets suitable for population studies. We found substantial genetic diversity among ancient horse Y chromosomal sequences, demonstrating that wild horses exhibited Y chromosomal diversity before domestication. The single 2,800-year-old domestic horse suggests that some level of Y chromosomal diversity still existed in domestic horses several thousands of years after domestication, although the lineage identified was closely related to the modern domestic lineage. These results clearly demonstrate both the feasibility and power of ancient Y chromosomal DNA sequence data to reveal past population processes and provide a more complete picture based on the history of both sexes. DNA extraction We extracted DNA from 90 ancient horse samples from Eurasia and North America ( Supplementary Table S2 ). To prepare the bone samples for extraction, we first cleaned the exterior surface of the bone using a Dremel tool to remove any potential surface contaminants. We then removed a 100–250 mg bone sample, which we pulverized with a mortar and pestle. We extracted DNA from the powder using the silica-based method described in ref. 39 . Primer design To investigate Y chromosome diversity in ancient and modern horses, we selected nine fragments within the noncoding regions of the Equus caballus Y chromosome reference sequence ( Supplementary Table S3 ). Five of these were first described in [9] . In addition to these five regions, we selected introns 1–3 of the amelogenin gene and the 3′ untranslated region of the SRY gene. All of those nine fragments were sequenced in 52 horses and the Przewalski horse [10] . Primer3 software ( http://frodo.wi.mit.edu/ [40] ).was used to design 88 primer pairs spanning the target region of ∼ 4 kb ( Supplementary Table S4 ). Each of these 88 fragments was then compared with the Horse Genome ( http://www.broadinstitute.org/mammals/horse [31] ) using a BLAT Search ( http://www.genome.ucsc.edu/cgi-bin/hgBlat [41] ). We excluded fragments that match with at least 50 bp and more than 80% identity to non Y chromosomal regions to reduce the probability of amplifying non Y chromosomal fragments of similar length and sequence. To test the multiplexing suitability and male-specific amplification of our primer set, we performed an initial PCR test using DNA from one modern male and female. PCR amplification and sequencing Immediately following extraction, we amplified one mitochondrial, one X-specific and one Y-specific fragment ( Supplementary Table S5 ) to test the extracts for DNA preservation and to identify male horses (Supplementary material sex test). On the basis of amplification success and on a selection strategy to optimize the geographic distribution of samples, we selected twelve samples for further analyses ( Supplementary Table S2 ). We used a two-step multiplex PCR [42] to amplify the 88 fragments ( Supplementary Table S4 ) from these 12 ancient samples. Extraction blanks were amplified for all of the 88 fragments to check for contamination. Further, all 88 fragments of each sample were amplified twice, starting from independent first step reactions, to detect potential DNA damage patterns. First-step PCR amplifications were performed in 25 μl reactions with 5 μl of DNA extract, 2 U AmpliTaq Gold DNA Polymerase and 1×buffer (Invitrogen), 1 mg ml −1 BSA (Sigma-Aldrich), 4 mM MgCl 2 , 250 μM of each dNTP, and 0.15 μM of each primer set (odd and even; Supplementary Table S3 ). Second-step PCR amplifications were performed in 25 μl reactions with 5 μl of 1:50 diluted first step PCR product, 0.1 U AmpliTaq Gold DNA Polymerase and 1×buffer (Invitrogen), 1 mg ml −1 BSA (Sigma-Aldrich), 4 mM MgCl 2 , 250 μM of each dNTP, and 1.5 μM of specific primer. The PCR thermal cycling conditions in the first-step multiplex PCR consisted of 95 °C for 12 min, followed by 35 cycles of denaturation at 94 °C for 20 s, annealing at 56 °C for 30 s and extension at 72 °C for 30 s, followed by a final extension at 72 °C for 4 min. For second-step PCR annealing temperatures, see Supplementary Table S4 . After second amplification, all extraction blank fragments and 16 (out of 88) randomly chosen fragments of each sample were loaded onto 2% agarose gels to test for clean controls and amplification success, respectively. Because the three non-permafrost horses chosen showed a low amplification success rate, for these samples, all 88 fragments were checked on a gel. The pattern of low success rate persisted, and these three samples were excluded from further processing. PCR products of the nine remaining samples ( Table 1 ) were purified using the Agencourt Ampure PCR purification kit, following the manufacturer's protocol, with some modifications that result in a fragment-length-specific cutoff during purification [43] . The purified products were quantified using a PicoGreen plate read on a Stratagene MX 3005P QPCR System. On the basis of this quantification, all 88 fragments per sample were normalized and pooled. The sample-specific fragment pools were barcoded for 454 high throughput sequencing using the methods described in [43] , [44] . After qPCR based quantification [45] , up to six barcoded sample-specific fragment pools (6×88 fragments) were sequenced on 1/16 of a 454 GS FLX run. 454 FLX Data processing and analysis Sequence reads were sorted based on their specific bar code using the program untag ( http://bioinf.eva.mpg.de/pts/ [43] ). Individual fragments were identified using demultiplex ( http://bioinf.eva.mpg.de/pts/ [43] ). Demultiplex searches for target primer sequences within untagged sequences, thereby identifying the reads. All reads containing the target specific 3′ and 5′ priming site and having a minimum of 85% identity to the reference were aligned to the target reference sequence. The consensus sequence for each fragment was called according to a 66% majority rule for all fragments, for which at least three reads per replicate were observed. The sequence data for both replicates from each sample were aligned, a consensus sequence was called and single fragments were merged, resulting in a total of 4,062 bp of sequence for each individual. For fragments with positions that differ in the two consensus replicates, we performed a third PCR, and a consensus sequence was called according to majority rule. Finally, an independent replication for all fragments containing polymorphic positions was performed in Copenhagen for the sample MGVo1_niche3.3. As all positions were replicated at least twice from independent PCR amplifications, we can rule out ancient DNA damage as a cause for any sequence variation observed among the obtained haplotypes. We then identified polymorphic positions based on a comparison of the complete 4,062 bp Y chromosome alignment of our nine ancient horses, the modern E. caballus and the E. przewalskii haplotypes ( Supplementary Table S3 ). We calculated a distance matrix showing the number of pairwise nucleotide differences among individuals using MEGA v4 ( http://www.megasoftware.net/ [46] ). We used DnaSP v5.10 to calculate nucleotide diversity (π) ( http://www.ub.es/dnasp/ [47] ). A median joining network was constructed using the software package Network 4.5. ( http://www.fluxus-engineering.com [48] ). As the ancient samples are from different time periods ( Table 1 ), we then tested for a correlation between the number of pairwise substitutions and the temporal differences between the 14 C dated samples to determine whether our diversity estimates were biased by age differences among the samples. We conducted a Spearman's rank correlation with P -values based on exact matrix permutation in R (version 2.10.0 [49] ). As the two samples associated with infinite radiocarbon ages (YG109.6, BL-O 728 ) could be incorrectly ranked, their minimum ages were switched and the test performed again. Using the Akaike information criterion implemented in MODELTEST 3.7 [50] , we identified GTR+I as the best fitting nucleotide substitution model for our alignment of the nine ancient horses and the three previously published Y chromosome sequences ( Supplementary Table S3 ). Bayesian phylogenetic and molecular clock analyses were then performed using BEAST v1.6.0 (refs 51 , 52 ) under the GTR+I model and assuming a strict molecular clock. To determine the best fitting coalescent model, marginal likelihoods were compared using Bayes Factors [53] between constant-size coalescent, an exponential growth, an expansion growth and a Bayesian skyline plot model, the latter allowing a flexible model of past population dynamics [54] ( Supplementary Table S6 ). For each analysis, we ran three MCMC chains of 10,000,000 iterations with trees and model parameter values sampled from the posterior distribution every 1,000th iteration. For each analysis, the first 10% were discarded from each run as burn-in, and the remainder combined. Convergence of the chains and effective sample sizes were verified using the program TRACER v1.5.0. The constant size model fit the data better than the more complex exponential growth and Bayesian skyline plot models and only marginally worse than the expansion growth model (log 10 BF: −0.053). As this is no decisive difference (decisive=log 10 BF >2 (ref. 55 )), the constant population size model was assumed to provide the best fit for the data. To estimate divergence times of the different haplotypes a final BEAST analysis was performed, in which evolutionary and coalescent model parameters were as for the best-fitting model above, but samples for which no radiocarbon date (JAL-292, JAL-310, MGVo1_niche3.3) or only a lower bound (infinite radiocarbon dates; BL-O 728 , YG 109.6) was available were also included by sampling their ages from a predefined distribution [56] . For the undated sequences, we sample from a lognormal distribution with 95% CIs between 600 and 80,000 years, and the weight of the sample density around 22,000 years. For the infinitely dated samples, the 95% CIs include the range 30,000–80,000 years, and the weight of the sample density is concentrated around 52,000 years. A further calibration was incorporated at the time of divergence between E. asinus , and the remaining lineages: We used a lognormal prior sampling between 1.0 and 5.5 myrs; these confidence intervals incorporate both the fossil record age estimates [57] , [58] , [59] and previous divergence estimates based on molecular data [60] . The results of the tip-dating analysis are shown in Supplementary Table S7 . Accession codes: All sequences have been deposited in nucleotide core GenBank database under the accession codes GQ495709 to GQ495789 . How to cite this article: Lippold, S. et al . Discovery of lost diversity of paternal horse lineages using ancient DNA. Nat. Commun. 2:450 doi: 10.1038/ncomms1447 (2011).